Activation and characterization of a cryptic polycyclic tetramate macrolactam biosynthetic gene cluster Polycyclic tetramate macrolactams (PTMs) are a widely distributed class of natural products with important biological activities. However, many of these PTMs have not been characterized. Here we apply a plug-and-play synthetic biology strategy to activate a cryptic PTM biosynthetic gene cluster SGR810-815 from Streptomyces griseus and discover three new PTMs. This gene cluster is highly conserved in phylogenetically diverse bacterial strains and contains an unusual hybrid polyketide synthase-nonribosomal peptide synthetase, which resembles iterative polyketide synthases known in fungi. To further characterize this gene cluster, we use the same synthetic biology approach to create a series of gene deletion constructs and elucidate the biosynthetic steps for the formation of the polycyclic system. The strategy we employ bypasses the traditional laborious processes to elicit gene cluster expression and should be generally applicable to many other silent or cryptic gene clusters for discovery and characterization of new natural products. Polycyclic tetramate macrolactams (PTMs) contain one tetramic acid and a polycyclic system (usually two to three rings) fused to macrolactams and exhibit diverse biological activities such as antifungal, antibiotic and antioxidant properties [1] , [2] , [3] , [4] , [5] , [6] , [7] . PTMs were previously isolated from symbionts of marine sponges, such as discodermide, alteramide A and cylindramide [5] . Recently, PTMs have been found in bacteria, such as maltophilin from Stenotrophomonas maltophilia [3] , heat-stable antifungal factor (HSAF) from Lysobacter enzymogenes [4] , [7] , as well as ikarugamycin [8] , dihydromaltophilin [2] and frontalamides [1] , all from medicinally important Streptomyces species. Most interestingly, Clardy and co-workers found that the PTM biosynthetic gene cluster from streptomycetes was a common origin for PTM biosynthesis in phylogenetically diverse bacteria and was conserved in more than 50% of the sequenced Streptomyces species [1] . Despite the emerging significance of PTMs in basic and applied biology, the mechanisms for the key steps in PTM biosynthesis such as installation of two polyketide chains and subsequent formation of the polycyclic system remain elusive [1] , [4] , [9] . One reason why the discovery and characterization of PTM biosynthetic gene clusters are challenging is because most of the PTM gene clusters remain silent under typical fermentation conditions either in the native or heterologous host. For example, after many trials, the frontalamide biosynthetic gene cluster was shown to become functional only under one specific culture condition [1] . Another obstacle is that most of the native producers are genetically intractable. As a matter of fact, these challenges are not unique to the PTM biosynthetic gene clusters. Numerous natural product biosynthetic gene clusters are considered as silent or cryptic [10] , [11] . A number of approaches has been developed to activate silent or cryptic biosynthetic gene clusters, such as manipulating cell culture parameters [12] , expressing the putative pathway-specific regulator under a well-characterized promoter [13] , testing a variety of heterologous hosts [14] or silencing other major secondary metabolite biosynthetic gene clusters [15] . However, these approaches can only be applied on a case-by-case basis. To discover and characterize novel PTM biosynthetic gene clusters, a generally applicable approach capable of activating cryptic gene clusters without specific tailoring to the gene cluster of interest is highly desirable. Here we use a simple synthetic biology strategy to activate the cryptic PTM biosynthetic gene cluster SGR810-815 from Streptomyces griseus and identify three putative PTMs. In addition, we elucidate their biosynthetic steps by creating and characterizing a series of gene deletion constructs. We not only confirm the iterative use of the single polyketide synthase-nonribosomal peptide synthetase (PKS-NRPS) module, but also provide new insights into the subsequent formation of the polycyclic system. Development of a gene cluster reconstruction system To discover and characterize new PTM biosynthetic gene clusters, we developed a simple synthetic biology strategy in which a plug-and-play scaffold is used to decouple gene cluster expression from native sophisticated regulation cascades ( Fig. 1 ). The key step in this strategy is to use a set of well-characterized promoters and the DNA assembler method [16] , [17] to reconstruct the target cryptic biosynthetic gene cluster in a genetically tractable heterologous host. The product(s) will be detected and characterized using analytical chemistry methods such as liquid chromatography-mass spectrometry (LC-MS) and NMR or biological activity assays. 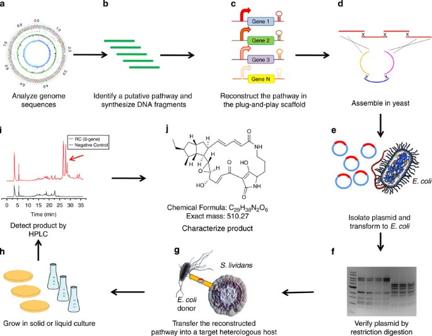Figure 1: The workflow of the synthetic biology strategy used to activate a cryptic biosynthetic gene cluster. Key steps include: (a) analysing a sequenced genome or metagenome to identify target biosynthetic gene clusters; (b) PCR-amplifying or chemically synthesizing the corresponding DNA fragments; (c) selecting a set of suitable promoters (well-characterized or newly identified according to the target heterologous host) for gene cluster reconstruction; (d) assembling the reconstructed biosynthetic gene cluster in yeast; (e) isolating the assembled constructs from yeast and re-transforming them intoE. colifor plasmid enrichment and verification; (f) verifying the assembled constructs by restriction digestion; (g) transferring the reconstructed biosynthetic gene cluster into the target heterologous host; (h) growing the strains in either liquid or solid media; (i) analysing samples on HPLC for product detection; (j) characterizing the potential products by LC-MS and NMR. Figure 1: The workflow of the synthetic biology strategy used to activate a cryptic biosynthetic gene cluster. Key steps include: ( a ) analysing a sequenced genome or metagenome to identify target biosynthetic gene clusters; ( b ) PCR-amplifying or chemically synthesizing the corresponding DNA fragments; ( c ) selecting a set of suitable promoters (well-characterized or newly identified according to the target heterologous host) for gene cluster reconstruction; ( d ) assembling the reconstructed biosynthetic gene cluster in yeast; ( e ) isolating the assembled constructs from yeast and re-transforming them into E. coli for plasmid enrichment and verification; ( f ) verifying the assembled constructs by restriction digestion; ( g ) transferring the reconstructed biosynthetic gene cluster into the target heterologous host; ( h ) growing the strains in either liquid or solid media; ( i ) analysing samples on HPLC for product detection; ( j ) characterizing the potential products by LC-MS and NMR. Full size image Because the DNA assembler method used for natural product gene cluster reconstruction relies on homologous recombination [16] , [17] , different promoters with low sequence similarity are needed for different genes in order to increase the gene cluster assembly efficiency. However, few constitutive or inducible promoters have been characterized in streptomycetes despite decades of research, and the reported commonly used promoter is ermE* p [18] , [19] , [20] . Therefore, promoter candidates upstream of 23 housekeeping genes originating from species in the Actinobacteria class were cloned and analysed. Thirteen promoters were highly active in Streptomyces lividans , and six of them were used in this study ( Supplementary Table S1 ). Activation of a cryptic PTM gene cluster As proof of concept, we sought to study an uncharacterized PTM gene cluster SGR810-815 from the sequenced S. griseus [21] . This gene cluster contains an evolutionarily conserved hybrid PKS-NRPS gene ( SGR814 ) with a size of approximately 9.5 kb. This PKS-NRPS gene contains DNA sequences encoding nine domains (KS-AT-DH-KR-ACP-C-A-PCP-TE) and is flanked upstream by a gene encoding a putative sterol desaturase and downstream by several putative oxidoreductase genes ( Supplementary Fig. S1a ). SGR814 shares 63% and 68% sequence identity with the PKS-NRPSs from the HSAF [7] and frontalamide [1] ( Fig. 2 ) biosynthetic gene clusters, respectively. 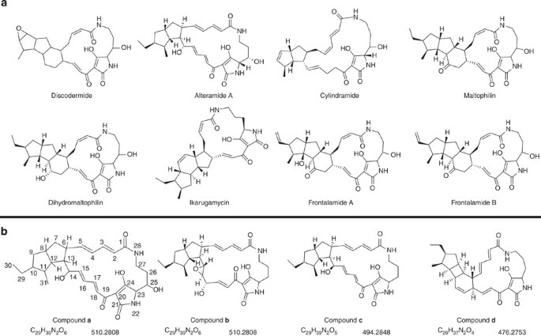Figure 2: The structures of PTM compounds. (a) Chemical structures of known PTMs. (b) Chemical structures of the products of the SGR810-815 gene cluster fromS. griseus. Note: the stereochemistry assignments of compoundb,c,dare relative. Figure 2: The structures of PTM compounds. ( a ) Chemical structures of known PTMs. ( b ) Chemical structures of the products of the SGR810-815 gene cluster from S. griseus . Note: the stereochemistry assignments of compound b , c , d are relative. Full size image We sought to reconstruct the entire gene cluster SGR810-815 by inserting six constitutive promoters upstream of the SGR genes (reconstructed cluster, Fig. 3a ). Two controls, one carrying the intact regulatory elements (original cluster) and the other containing the ermE* p promoter added upstream of the whole cluster (Ep), were also constructed ( Supplementary Fig. S1b and Supplementary Table S2 ). The gene fragments and the promoter fragments were PCR amplified and assembled using the DNA assembler method [17] and the correct constructs were verified by restriction digestions. All these constructs were integrated into S. lividans for heterologous expression. As shown in Fig. 3b , all the genes in the reconstructed gene cluster were substantially transcribed, and the first gene under the rpsL p ( Cellulomonas flavigena ) promoter showed an approximately 150-fold higher expression level compared with the internal control hrdB [22] , [23] , [24] . In contrast, the expression levels for most SGR genes in either the native producer ( S. griseus , SG) or two control strains were very low. These data confirmed the silencing of the gene cluster under the typical cultivation conditions, and suggest that via gene cluster reconstruction, the transcription of each gene in a cryptic gene cluster could be significantly increased. We then extracted the metabolites from the S. lividans strain harbouring the reconstructed SGR810-815 gene cluster and performed high-performance liquid chromatography-MS (HPLC-MS) analysis. The reconstructed gene cluster produced two major products and three minor products compared with the negative control ( S. lividans without the target gene cluster; Fig. 3c ). The potential product peaks were observed at around 26–28 min with the same corresponding mass of [M+H] + =511. 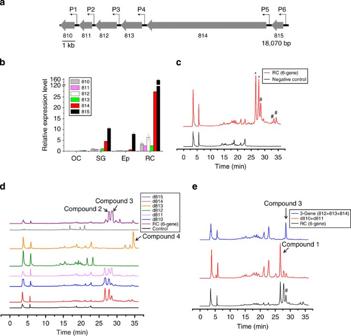Figure 3: Activation and characterization of a cryptic PTM gene cluster. (a) The reconstructed cryptic SGR810-815 gene cluster fromS. griseus. P1: gapdh(Kocuria rhizophila), P2: gapdh(S. griseus), P3: ermE*, P4: rpsL(Tsukamurella paurometabola), P5: rpsL(S. griseus), P6: rpsL(Cellulomonas flavigena). (b) Real-time PCR analysis of SGR genes in the reconstructed gene cluster and the control gene clusters. Ep, original cluster with ermE*p in front of the whole gene cluster; OC, original cluster; SG, native producerS. griseus; RC, reconstructed cluster. Error bars represent the standard errors and triplicates were performed for each reaction. (c) HPLC analysis of the extract from theS. lividansstrain carrying the reconstructed gene cluster SGR810-815. *Major products, #minor products. Ultraviolet chromatographs were recorded at 260 nm. (d) HPLC analysis of single-deletion constructs. (e) HPLC analysis of three-gene and four-gene constructs (# indicates a small production of compoundc). Figure 3: Activation and characterization of a cryptic PTM gene cluster. ( a ) The reconstructed cryptic SGR810-815 gene cluster from S. griseus . P1: gapdh( Kocuria rhizophila ), P2: gapdh( S. griseus ), P3: ermE*, P4: rpsL( Tsukamurella paurometabola ), P5: rpsL( S. griseus ), P6: rpsL( Cellulomonas flavigena ). ( b ) Real-time PCR analysis of SGR genes in the reconstructed gene cluster and the control gene clusters. Ep, original cluster with ermE*p in front of the whole gene cluster; OC, original cluster; SG, native producer S. griseus ; RC, reconstructed cluster. Error bars represent the standard errors and triplicates were performed for each reaction. ( c ) HPLC analysis of the extract from the S. lividans strain carrying the reconstructed gene cluster SGR810-815. *Major products, #minor products. Ultraviolet chromatographs were recorded at 260 nm. ( d ) HPLC analysis of single-deletion constructs. ( e ) HPLC analysis of three-gene and four-gene constructs (# indicates a small production of compound c ). Full size image Isolation and characterization of putative PTMs To determine the chemical structures of these compounds, large-scale cultivation on solid plates (equivalent to ~4 l liquid culture) of the heterologous host harbouring the target reconstructed gene cluster was carried out to obtain sufficient amounts of these compounds. High-resolution electrospray ionization mass spectrometry in positive mode showed an m/z of 511.2807 for compound a [M(C 29 H 38 O 6 N 2 )+H] + (calculated: 511.2808) and 511.2781 for compound b [M(C 29 H 38 O 6 N 2 )+H] + (calculated: 511.2808). Their corresponding chemical structures ( Fig. 2b ) were elucidated by extensive one- and two-dimensional NMR spectroscopy ( 1 H, 13 C, Double-Quantum Filtered Correlation spectroscopy (COSY), Total correlation spectroscopy (TOCSY), Heteronuclear single-quantum correlation spectroscopy (gHSQC), Heteronuclear multiple-bond correlation spectroscopy (gHMBC) and Nuclear Overhauser Effect Spectroscopy (NOESY)) and MS experiments ( Supplementary Figs S2–S4 , Supplementary Table S3 ). Key COSY and heteronuclear multiple bond correlation (HMBC) correlations were summarized in Supplementary Fig. S5 . For compound a , the Double-Quantum Filtered COSY (Phase-sensitive) spectrum revealed the spin system, and the HMBC supported the coupling of H2 and H3 to C1, as well as H23 to C19. For compound b , the characteristic C-H coupling constants (C14, J C-H =172 Hz and C15, J C-H =181 Hz, measured using a high-resolution coupled gHSQC) suggested the presence of an epoxide ring [25] . All compounds belong to the group of tetramic acid-containing macrolactam natural products. Compound a shares the same structure as previously reported alteramide A [26] , whereas compound b has never been reported in literature. The NOESY correlations to confirm the stereochemistry of compound b were summarized in Supplementary Fig. S6 . The production of these tetramic acid-containing macrolactams in a heterologous host clearly confirms the iterative use of the single PKS-NRPS module, which is rare in bacteria. Moreover, we have cultivated the previously described control strains and the native producer S. griseus under multiple different cultivation conditions (MYG liquid or solid media and YMS liquid or solid media), and the fermentation broths were extracted and analysed by HPLC. For the control strains, no distinct difference was observed compared with the wild-type S. lividans . For the native producer, neither compound a nor compound b could be detected. Elucidation of the biosynthetic steps Next, we attempted to elucidate the biosynthetic steps of this new gene cluster using the same synthetic biology strategy. We first determined the exact boundary of the gene cluster by bioinformatics analysis of upstream and downstream regions of this gene cluster and then constructed another seven-gene gene cluster with an upstream putative aminotransferase gene ( Supplementary Fig. S7a and Supplementary Table S4 ). The expression of this putative aminotransferase gene was confirmed by quantitative PCR and the products were identified to be the same as the ones from the six-gene gene cluster ( Supplementary Fig. S7b ), indicating that the putative aminotransferase gene was not essential. Then, to decipher the biosynthetic steps, a series of mutant gene clusters consisting of single or multiple gene deletions were constructed and analysed ( Fig. 3d and e , Supplementary Tables S5 and S6 , Supplementary Figs S8 and S9 ). As expected, the SGR814 single-deletion construct lost the ability to produce any target compounds, indicating the essential role of the PKS-NRPS hybrid gene ( Fig. 3d ). The SGR815 single-deletion construct ( Fig. 3d ) abolished the production of compound a and instead produced compound c [M(C 29 H 38 O 5 N 2 )+H] + with an m/z of 495.2864 ( Fig. 2b and Supplementary Figs S5, S6, S10 and S11 , Supplementary Table S7; calculated: 495.2859). Compound c shares the similar structure as the previously reported alteramide A [26] except for the lack of one hydroxyl group and the different stereochemistry of carbon 14. By comparing the structures of compound a and compound c , we noticed that the difference is the lack of a hydroxyl group proximal to the tetramic-acid moiety of the compounds. Therefore, it was clear that SGR815 serves as a hydroxylase, similar to its homologous enzyme characterized in the HSAF [27] and frontalamides [1] gene clusters. Both the SGR812 single-deletion construct and the SGR814 single-gene construct (the construct only contains the SGR814 gene under a strong constitutive promoter) failed to produce any related compounds, indicating that SGR812 may be involved in the first step of the formation of the polycyclic system ( Fig. 3d ). The SGR813 single-deletion construct ( Fig. 3d ) revealed one major peak at ~34 min with a corresponding m/z of 477.2757 for compound d [M(C 29 H 36 O 4 N 2 )+H] + (calculated: 477.2753) and the chemical structure of compound d was subsequently determined ( Fig. 2b , Supplementary Figs S5, S6, S10 and S12 , Supplementary Table S7 ). The interesting four-membered ring in compound d is the first observation of such structure in known PTMs. The structure of compound d suggests that it may be a shunt product after SGR813 deletion. These results suggest that both SGR812 and SGR813 are involved in the formation of the polycyclic system. To further confirm this, a three-gene gene cluster consisting of SGR812, SGR813 and SGR814 was constructed and evaluated ( Supplementary Fig. S9 ). Compound c was found to be the major product ( Fig. 3e ), indicating that this compound is a key biosynthetic intermediate. In addition, a four-gene gene cluster consisting of SGR812, SGR813, SGR814 and SGR815 was constructed ( Supplementary Fig. S9 ) and its main product was compound a ( Fig. 3e ), which again confirmed the functional roles of these four genes. Although the SGR810 and SGR811 single-deletion constructs both maintained the production of compound a and compound b , the loss of compound b in these three-gene and four-gene constructs indicates that SGR810 and SGR811 are involved in the formation of the epoxide ring and their functions might be redundant ( Fig. 3d and e ). Taken together, a biosynthetic route for this group of PTMs has been proposed ( Fig. 4 ). 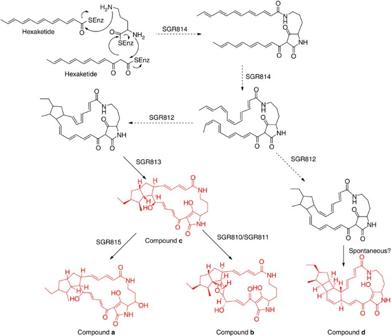Figure 4: Proposed biosynthetic mechanism for formation of the four tetramic acid-containing macrolactams. The PKS is responsible for the hexaketide chain synthesis and works together with the NRPS to condense the two polyketide chains with ornithine. The formation of the first polycyclic ring is catalysed by SGR812 and the second ring is closed by SGR813. Compoundcis the key intermediate that can be converted into compoundaby SGR815 or compoundbby SGR810/SGR811. A shunt product compounddwill be formed if SGR813 is absent in the cluster. SEnz is the carrier protein within the PKS or NRPS. The red structures are the ones with full set of NMR data. Figure 4: Proposed biosynthetic mechanism for formation of the four tetramic acid-containing macrolactams. The PKS is responsible for the hexaketide chain synthesis and works together with the NRPS to condense the two polyketide chains with ornithine. The formation of the first polycyclic ring is catalysed by SGR812 and the second ring is closed by SGR813. Compound c is the key intermediate that can be converted into compound a by SGR815 or compound b by SGR810/SGR811. A shunt product compound d will be formed if SGR813 is absent in the cluster. SEnz is the carrier protein within the PKS or NRPS. The red structures are the ones with full set of NMR data. Full size image We have successfully activated a silent PTM gene cluster and discovered three novel PTM compounds by fully reconstructing the target gene cluster in a heterologous host. The production of these novel tetramic acid-containing macrolactams in a heterologous host directly confirms the iterative use of the single PKS-NRPS module, which is an intriguing feature of this type of enzymes in bacteria. Although this cluster shares sequence homology with other characterized PTM gene clusters and the PTMs characterized from these gene clusters all share similar backbones, there are notable differences in their chemical structures. There are basically two different groups of PTMs, one with a 5,5,6-tricyclic system or 5,6,5-tricyclic system fused to the macrolactam and the other with a 5,5-bicyclic system ( Fig. 2 ). It appears that the products we have discovered belong to the second group. It should be noted that these products may be shunt products from the gene cluster because of heterologous expression, but the different structures still reveal the diversity of PTMs. In addition, we used the same synthetic biology strategy to investigate the biosynthetic route, especially for the formation of the polycyclic system. SGR815 was confirmed to be a hydroxylase, which is conserved in all known PTM gene clusters. SGR812 and SGR813 were annotated as oxidoreductases and can be found in most of the known PTM gene clusters. Based on phylogenetic analysis, these two enzymes are distinct and may catalyse different reactions even though they belong to the same family of oxidoreductases. Indeed, our results from the gene deletion constructs suggest that SGR812 is involved in the formation of the first ring, whereas SGR813 is responsible for the closure of the second ring. Interestingly, we noticed that two related PTM gene clusters from Saccharophagus degradans and Salinospora arenicola only contain homologs of SGR812, which supports the proposed role of SGR812 in ring formation. That is because the reaction catalysed by SGR812 takes place before the ones catalysed by other oxidoreductases. The last two enzymes, SGR811 and SGR810, are also conserved in most of the related PTM gene clusters, but with greater sequence diversity. Our results suggest that they are likely to perform oxidative reactions on the backbone. It should be noted that the strategy we employed in this study is simple, generally applicable and potentially scalable in studying other cryptic natural product gene clusters. For example, we recently used the same strategy to successfully reconstruct a putative phosphonic acid gene cluster from a Streptomyces sp. soil isolate. Analysis of the S. lividans strain containing the completely reconstructed 13-gene pathway revealed multiple new putative phosphonate peaks by 31 P-NMR, which were not observed in the native host or the S. lividans background ( Supplementary Fig. S13 ). The key innovative aspect of this strategy is the use of the DNA assembler method to achieve full gene cluster reconstruction for cryptic gene clusters in a single-step manner. This strategy is distinct from other related strategies such as using promoter replacement to activate cryptic single genes [28] , which focuses on single genes rather than the entire gene cluster, gene-by-gene reassembly in a heterologous host [29] , [30] , [31] , which use multiple plasmids to reconstruct known gene clusters or perform the assembly in multiple steps, or use of recombination-based systems for gene cluster activation [32] , which directly clone an entire gene cluster without any reconstruction. Using the same experimental set-up, this strategy can in principle enable the activation of many cryptic PTM biosynthetic gene clusters of interest in streptomycetes and other actinomycetes. Moreover, this strategy may be further modified for activation of cryptic gene clusters from other organisms, such as myxobacteria, cyanobacteria and fungi, as long as appropriate heterologous hosts and functional promoters can be obtained. For the promoters, strong constitutive promoters used to drive the expression of each gene in a target gene cluster can be readily identified from the heterologous host by real-time PCR or RNA-seq. It is noteworthy that because of the plug-and-play nature of the system, a cryptic gene cluster of interest can be readily reconstructed and the entire process may be fully automated. Our long-term goal is to build an automated, scalable and high-throughput platform for natural product discovery. Utilizing an integrated robotic system featuring liquid handler with Peltier blocks (setting up PCR reactions, isolating plasmid DNAs, DNA transformation in S. cerevisiae and S. lividans ), thermal cyclers (synthesis of DNA fragments by PCR reactions), magnetic bead separator (DNA purification), shake incubators (cell cultivation) and LC-MS (compound detection), this versatile platform will be capable of assembling and reconstruction hundreds of gene clusters per day with minimal human intervention. With the continually decreasing cost of DNA synthesis, the entire gene cluster may be reconstructed by using synthetic genes and/or promoters. Finally, this strategy is much more flexible and versatile for generating gene deletions or additions for mechanistic studies or creation of novel compounds than traditional combinatorial biosynthesis approaches. Overall, the synthetic biology approach we developed represents a new technology platform for discovery and characterization of novel natural products from sequenced genomes and metagenomes for pharmaceutical and biotechnological applications. Materials and reagents S. lividans 66 and S. griseus were obtained from the Agricultural Research Service Culture Collection (Peoria, IL, USA). The vector map and complete sequences of Streptomyces integration parts of plasmid pAE4 (ref. 33 ) is provided in Supplementary Fig. S14 . E. coli strain WM1788 is the equivalent of strain BW25141 (ref. 34 ) [ lacI q rrnB T14 Δ lacZ WJ16 Δ phoBR580 hsdR514 Δ araBAD AH33 Δ rhaBAD LD78 galU95 endA BT333 uidA (Δ Mlu I):: pir + recA1 , derived from E. coli K-12 strain BD792] and was provided by Dr William Metcalf (University of Illinois, Urbana, IL, USA). E. coli strain WM6026 (refs 35 , 36 ) [ lacI q rrnB3 Δ lacZ 4787 hsdR514 Δ araBAD567 Δ rhaBAD568 rph-1 att l::pAE12(Δ ori R6K- cat ::Frt5) Δ endA ::Frt uidA (ΔMluI):: pir att HK::pJK1006Δ( ori R6K- cat ::Frt5; trfA ::Frt)] was provided by Dr William Metcalf (University of Illinois, Urbana, IL, USA). The plasmid pRS416 was purchased from New England Biolabs (Beverly, MA). Nalidixic acid and isopropyl-β- D -thiogalactopyranoside were obtained from Sigma-Aldrich (St Louis, MO). ISP2, agar, beef extract, yeast extract, malt extract and other reagents required for cell culture were obtained from Difco (Franklin Lakes, NJ). All restriction endonucleases, as well as T4 DNA ligase and antarctic phosphatase, were purchased from New England Biolabs (Beverly, MA). Phusion DNA polymerase was from Finnzymes (Waltham, MA). Failsafe PCR 2 × PreMix G was purchased from EPICENTRE Biotechnologies (Madison, WI), which was used as the buffer to amplify gene cluster fragments. SYBR Green PCR Master Mix was purchased from Applied Biosystems (San Francisco, CA). The QIAprep Spin Plasmid Mini-prep Kit, QIAquick PCR Purification Kit, QIAquick Gel Extraction Kit and RNeasy MinElute Cleanup Kit were purchased from Qiagen (Valencia, CA). All primers were synthesized by Integrated DNA Technologies (Coralville, IA). Yeast YPAD medium-containing 1% yeast extract, 2% peptone and 2% dextrose supplemented with 0.01% adenine hemisulphate was used to grow S. cerevisiae HZ848 ( MAT α, ade 2-1, Δ ura 3, his 3-11, 15, trp 1-1, leu 2-3, 112 and can 1-100), which was used as the host for DNA assembly. Synthetic complete drop-out medium lacking uracil (SC-Ura) was used to select transformants containing the assembled biochemical gene clusters of interest. Streptomycete cultivation and expression analysis A seed culture was grown in MYG medium (10 g l −1 malt extract, 4 g l −1 yeast extract and 4 g l −1 glucose) at 30 °C with constant shaking (250 r.p.m.) until saturation, and inoculated into fresh MYG with a ratio of 1:100. The total RNA was extracted using the RNeasy Mini Kit (Qiagen). Reverse transcription was carried out using the First-strand cDNA Synthesis Kit (Roche Applied Science, Indianapolis, IN). Real-time PCR was performed with SYBR Green PCR Master Mix on the 7900HT Fast Real-Time PCR System (Applied Biosystems, Carlsbad, CA). Primers were designed by the online tool provided by Integrated DNA Technologies ( https://www.idtdna.com/scitools/Applications/RealTimePCR/ ). 10 μl of 2 × SYBR Green Mix, 1 μl of cDNA, 1 μl of each primer at a concentration of 10 pmol μl −1 and 7 μl of ddH 2 O were mixed gently in each well of the Applied Biosystems MicroAmp Optical 96-Well Reaction Plate. Reactions were performed using the following programme: 2 min at 50 °C, 10 min at 95 °C for one cycle followed by 15 s at 95 °C, 30 s at 60 °C and 30 s at 72 °C for 40 cycles with a final cycle of 10 min at 72 °C. The endogenous gene hrdB , encoding RNA polymerase sigma factor, was used as the internal control for promoter screening. The expression levels of other candidate genes were normalized by the expression of the control. Data were analysed using SDS2.4 software (Applied Biosystems). Gene cluster reconstruction and yeast transformation Gene cluster fragments were amplified from the genomic DNA of S. griseus . The primer sequences are listed in Supplementary Tables S2–S5 . The S. cerevisiae helper fragment was amplified from the plasmid pRS416, whereas the E. coli helper fragment and the S. lividans helper fragment were amplified from pAE4. The PCR products were individually gel-purified from 0.7% agarose. For gapdh p (SG) and rpsL p (SG), the genomic DNA of S. griseus was isolated using the Wizard Genomic DNA Purification Kit (Promega, Madison, WI) and then used as the template for PCR amplification of the two target promoters. Promoters from other hosts were obtained through primer splicing in which six to ten overlapping oligonucleotides designed based on the sequence of each promoter are joined together by overlap extension PCR. Genes with corresponding promoters were also ligated together by overlap extension PCR. To ensure high efficiency of yeast homologous recombination, the ‘promoter upstream-gene-promoter downstream’ cassette was built to generate a ~200-bp overlap region with adjacent fragments. Individual cassettes (200–300 ng of each) were mixed and precipitated with ethanol. The resulting DNA pellet was air-dried and resuspended in 4 μl of Milli-Q double deionized water. The concentrated mixture of DNA was electroporated into S. cerevisiae using the protocol reported elsewhere [16] , [17] . Restriction digestion analysis Colonies were randomly picked to SC-Ura liquid media and grown for 1 day, after which the plasmids from yeast were isolated using Zymoprep II Yeast Plasmid Miniprep kit (Zymo Research, CA). Yeast plasmids were transformed to E. coli strain BW25141 and selected on Luria Broth (LB) agar plates supplemented with 50 μg ml −1 apramycin. Colonies were inoculated into 5 ml of LB media supplemented with 50 μg ml −1 apramycin, and plasmids were isolated from the liquid culture. Plasmids isolated from E. coli were then subjected to restriction digestion. Usually, three enzymes cutting the target molecule at multiple sites were chosen. The reaction mixtures were loaded to 1% agarose gels to check for the correct restriction digestion pattern by DNA electrophoresis ( Supplementary Fig. S15 ). For the original and fully reconstructed gene clusters, an efficiency of 30–40% was achieved for DNA assembly. For all the deletion constructs, 60%, 70%, 70%, 60%, 100% and 40% efficiencies were achieved for deletion of SGR810, SGR811, SGR812, SGR813, SGR814 and SGR815, respectively. Heterologous expression in S. lividans The verified clones were transformed to E. coli WM6026 (ref. 35 ) and selected on LB agar plates supplemented with 19 μg ml −1 2,6-diaminopimelic acid and 50 μg ml −1 apramycin. These transformants were then used as the donors for conjugative transfer of the assembled plasmids to S. lividans 66 following the protocol described elsewhere [35] . S. lividans exconjugants were picked and re-streaked on ISP2 plates supplemented with 50 μg ml −1 apramycin and grown for 2 days. For the reconstructed gene cluster SGR810-815, a single colony was inoculated into 20 ml of ATCC172 liquid medium (5 g l −1 yeast extract, 20 g l −1 soluble starch, 5 g l −1 N-Z Amine Type A, 1 g l −1 CaCO 3 and 10 g l −1 glucose) supplemented with 50 μg ml −1 apramycin in a 125-ml shake-flask (3 mm glass beads added to improve liquid mixing and aeration). Aliquots of this seed culture with a volume of 250 μl were spread for confluence over Petri plates containing approximately 25–30 ml of YMS solid agar medium (4 g l −1 yeast extract, 10 g l −1 malt extract, 4 g l −1 soluble starch and 20 g l −1 Bacto agar) and the plates were incubated for 7 days at 30 °C. HPLC-MS analysis To isolate potential compounds, agar and the adherent cells were stored at −80 °C for 24 h, after which the frozen cultures were thawed completely and the released liquids were collected. The liquids were extracted by ethyl acetate with a ratio of 1:1 twice, concentrated 1,000-fold and subjected to HPLC analysis. HPLC was performed on the Agilent 1100 series LC/MSD XCT plus ion trap mass spectrometer with a Phenomenex Luna C18 reverse-phase column (3.0 × 150 mm 2 , 3.5 μm). HPLC parameters were as follows: solvent A, 0.1% formic acid in water; solvent B, 0.1% formic acid in acetonitrile; gradient, 10% B for 5 min, to 100% B in 25 min, maintain at 100% B for 10 min, return to 10% B in 1 min and finally maintain at 10% B for 9 min; flow rate 0.3 ml min −1 ; detection by ultraviolet spectroscopy at 260 nm. Under such conditions, products are eluted at 26.8 min (compound a ), 27.8 min (compound b ), 28.5 min (compound c ) and 34.6 min (compound d ). The MS system was operated using a drying temperature of 350 °C, a nebulizer pressure of 35 p.s.i., a drying gas flow of 8.5 l min −1 and a capillary voltage of 4,500 V. Structure elucidation of compounds a–d Compounds a , b , c and d were isolated by reverse-phase HPLC using a Phenomenex Luna 10u C18 column (10 × 250 mm 2 ), on the Agilent 1100 series LC/MSD XCT with an isocratic solvent of 60% acetonitrile in water with 0.1% formic acid (with a flow rate of 3 ml min −1 and a wavelength of 260 nm). The high-resolution MS was performed on a Waters Q-Tof Ultima system (Walters, Milford, MA). All NMR experiments were carried out on a Varian UNITY INOVA 600 MHz spectrometer, except the 13 C spectra, which were recorded on a Bruker Avance III 500i with a 5 mm 13 C( 1 H) cryogenic probe at the National Magnetic Resonance Facility at the University of Wisconsin at Madison. The structures were determined based on 1-D and 2-D NMR data. The relative configurations were determined by using 2-D NOESY experiments. How to cite this article: Luo, Y. et al. Activation and characterization of a cryptic polycyclic tetramate macrolactam biosynthetic gene cluster. Nat. Commun. 4:2894 doi: 10.1038/ncomms3894 (2013).